High-throughput detection of miRNAs and gene-specific mRNA at the single-cell level by flow cytometry Fluorescent in situ hybridization (FISH) is a method that uses fluorescent probes to detect specific nucleic acid sequences at the single-cell level. Here we describe optimized protocols that exploit a highly sensitive FISH method based on branched DNA technology to detect mRNA and miRNA in human leukocytes. This technique can be multiplexed and combined with fluorescent antibody protein staining to address a variety of questions in heterogeneous cell populations. We demonstrate antigen-specific upregulation of IFNγ and IL-2 mRNAs in HIV- and CMV-specific T cells. We show simultaneous detection of cytokine mRNA and corresponding protein in single cells. We apply this method to detect mRNAs for which flow antibodies against the corresponding proteins are poor or are not available. We use this technique to show modulation of a microRNA critical for T-cell function, miR-155. We adapt this assay for simultaneous detection of mRNA and proteins by ImageStream technology. Single-cell analysis is a rapidly growing field in biomedical research that yields an unprecedented level of information [1] , [2] . Flow cytometry has been the gold standard for high-throughput phenotypic and functional characterization of various cell types. While the major advantages of flow cytometry include a simple workflow using fluorescently labelled antibodies for the detection of intracellular or surface markers and high throughput, this technology is limited by availability of highly specific and sensitive reagents for antigens. Advances in molecular biology have enabled techniques such as microarrays, quantitative PCR and RNA sequencing [3] , [4] , [5] . These technologies are sequence based and not constrained by antibody availability, providing ‘unrestricted’ tools for in-depth analysis of transcriptional signatures that define cell functions in physiologic or disease states. The major drawback of most of these approaches is the generation of transcriptional signatures in bulk populations of cells, which may provide insufficient and/or spurious information on the biologic entity of rare subsets within heterogeneous populations [6] . More recently, new methods such as microfluidic platforms and adaptations of RNAseq have been successfully used for single-cell transcriptional analysis [7] , [8] . However, for these techniques, single cells must to be first live sorted and the laborious methods required to isolate and amplify RNA can result in a significant loss of RNA species [9] . Fluorescent in situ hybridization (FISH) is another method used for the detection of specific nucleic acid sequences at the single-cell level [10] . It is based on fluorescently labelled probes and has been widely used in fluorescence microscopy to detect RNA or DNA sequences in cells adhered to coverslips or tissues [11] . Even though this powerful imaging technique enables detection of down to a single copy of a given nucleic acid sequence [12] and simultaneous analysis of intracellular structures and localization, it has so far been poorly adaptable to flow cytometry. Flow cytometric identification of RNA species would have several major comparative advantages. Whereas microscopy is practically limited to analysis of a few hundred cells, flow cytometry allows high-throughput acquisition of up to millions of cells in a single sample and combination of larger varieties of fluorescent channels; acquisition of 10–15 fluorescent markers are now routinely performed on four- or five-laser cytometers. Several adaptations of microscopy methods have been attempted in the past to detect FISH signals with flow cytometry [13] , [14] , [15] . However, they were limited to nucleic acid sequences with abundant expression, such as viral RNAs after acute infection [14] . More recently, another study [16] achieved detection of lower levels of RNA and oncogene expression in cell lines, and identified viral genes (that is, human immunodeficiency virus (HIV)) after in vitro infection of primary samples. Another limitation of previous experimental approaches is the inability to combine mRNA detection with antibody staining of proteins, a critical tool to define specific cell subsets in mixed populations. Here we describe a novel flow-FISH method for high-throughput detection of mRNA and microRNA (miRNA). This method is derived from the QuantiGene ViewRNA FISH cell assay (RNA-FISH) that was developed by Affymetrix for microscopy [17] . We show here that new protocols developed in our laboratory, when used in combination with this technique, enable the simultaneous detection of several mRNA molecules in various leukocyte subsets from human blood identified by antibody staining of cell surface markers. We demonstrate sensitive and specific detection of cytokines such as interferon-γ (IFNγ) and interleukin (IL)-2 mRNA of HIV- and cytomegalovirus (CMV)-specific CD4 and CD8 T cells. We confirm specificity of cytokine mRNA detection by simultaneous IFNγ mRNA-FISH and IFNγ protein secretion capture assays. We highlight the ability of this assay to overcome the limitation of antibody availability by excellent detection of IL-21, a cytokine for which intracellular cytokine staining (ICS) with a fluorescent antibody is not sensitive enough to allow adequate quantitation. Furthermore, we use this assay to detect the expression of Indoleamine 2,3-Dioxygenase (IDO), an enzyme for which no flow cytometry antibody was available at the time these experiments were performed. Similarly, we show that this technique can be readily used for the detection of small miRNA molecules that play major regulatory roles in eukaryotic cells without being translated into proteins. Finally, we prove that this approach can be used in combination with ImageStream technology, allowing for high-throughput subcellular compartmentalization studies of mRNA and protein co-expression. Taken together, these results show the power and high versatility of this novel technology to address biomolecular mechanisms in heterogeneous cell populations. Detection of mRNA and antibody staining by flow cytometry One of the major limitations of typical FISH protocols is the variable requirement in hybridization times and conditions for different probe sets. In contrast, a specific algorithm is used for the QuantiGene ViewRNA method that allows for the design of probes that exhibit high sensitivity and specificity as well as the same hybridization temperature. This provides greater reproducibility between different probes and experimental designs and facilitates assay multiplexing. A prerequisite for the use of this technology in flow cytometry is the availability of hybridization and staining reagents compatible with cells in suspension. Initial testing revealed that cell buoyancy and cell lysis were major issues with the buffers developed for adherent cells and fluorescent microscopy, resulting in massive subsequent cell loss ( Supplementary Fig. 1 ). Even though we were still able to reliably detect 18 s ribosomal RNA with flow cytometry, such a large cell loss, along with the incompatibility between the initial FISH protocol and antibody staining, made this protocol unfavourable for the analysis of primary cells in general and rare subpopulations, such as antigen-specific T cells in particular. Through a collaborative effort, we therefore developed alternative methods to process non-adherent cells. The cells were fixed with a methanol-based reagent before permeabilization. This new protocol was less harsh to the cells, leading to reduced cell loss and preservation of the main morphologic characteristics as indicated by forward and side scatter ( Fig. 1a,b ). We next performed head-to-head comparison of antibody staining using a standard surface stain flow cytometry protocol or the new flow-RNA assay. To this purpose, we selected fluorochromes resistant to methanol fixation [18] that stained for surface markers identifying main peripheral blood mononuclear cell (PBMC) subsets. In our hands, Brilliant Violet, Alexa and eFluors dyes perform particularly well. We assessed the respective ability of specific antibody clones to recognize epitopes that withstand the procedures. As previously reported, the potential usability of an antibody depends on both the protein targeted and the specific clone. Although several manufacturers provide useful references as to which reagents are suitable with methanol-based flow protocols, in our experience this use still requires careful assessment by the investigator for each specific mRNA flow-FISH application. Once we had identified appropriate combinations, surface staining for PBMC subsets combined with the Flow-RNA assay gave excellent results, with definition of cell populations very similar to a standard flow cytometry protocol ( Fig. 1a,b ). Furthermore, the new buffer used is compatible with dead cell viability dyes ( Fig. 1b ). 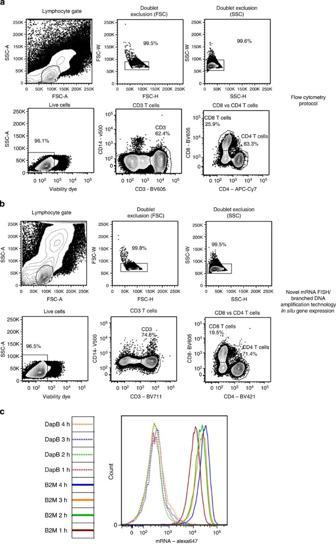Figure 1: Antibody staining and detection of housekeeping genes. Comparison of physical and phenotypic characteristics of PBMCs stained with a dead cell dye and fluorescent antibodies for CD3, CD4, CD8 and CD14 using either (a) a standard surface stain flow cytometry protocol or (b) the new flow-RNA assay (representative out of five). (c) Kinetic experiment of different hybridization incubation times following staining with either an irrelevant probe for the bacterial gene DapB or the housekeeping gene β2M (representative example out of three). Figure 1: Antibody staining and detection of housekeeping genes. Comparison of physical and phenotypic characteristics of PBMCs stained with a dead cell dye and fluorescent antibodies for CD3, CD4, CD8 and CD14 using either ( a ) a standard surface stain flow cytometry protocol or ( b ) the new flow-RNA assay (representative out of five). ( c ) Kinetic experiment of different hybridization incubation times following staining with either an irrelevant probe for the bacterial gene DapB or the housekeeping gene β2M (representative example out of three). Full size image The mRNA probes have optimal hybridization temperature of about 40 °C. To identify the hybridization time that confers optimal signal-to-noise ratio for detection, we performed a kinetics experiment using either an irrelevant probe towards DapB (dihydopicolinate reductase of Bacillus subtilis) or a probe specific for the housekeeping mRNA β2-microglobulin (β2M). A plateau was reached between the 2- and 4-h hybridization times ( Fig. 1c ), with excellent signal-to-noise ratio. We thus selected the 2-h hybridization step for subsequent experiments. A schematic representation of the workflow can be found in Fig. 2 . 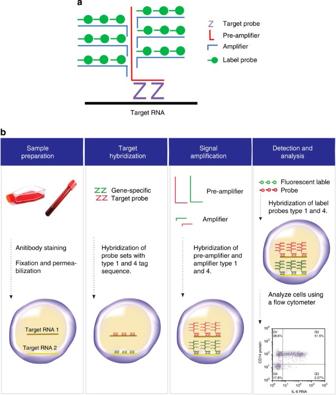Figure 2: Schematic representation of Flow-FISH methodology (a) Structure of target probe hybridization with the amplifying branched DNA sequences and the label DNA probes. (b) Diagram representing the workflow of the flow-FISH assay. Figure 2: Schematic representation of Flow-FISH methodology ( a ) Structure of target probe hybridization with the amplifying branched DNA sequences and the label DNA probes. ( b ) Diagram representing the workflow of the flow-FISH assay. Full size image The sensitivity of the assay varies depending on the probes used (as different probes have different affinities) and the target sequence of interest (small RNA sequences are targeted by fewer probes resulting in potentially weaker signal). On the basis of our preliminary data shown in Supplementary Fig. 2 , we can confidently detect about 10 mRNA copies per cell for the housekeeping gene HMBS (hydroxymethylbilane synthase). It is recommended that users should perform their own validation to identify the sensitivity of the assay based on the target of interest, the cell type and the specific experimental design. Sequences of the probes used in our studies are detailed in Supplementary Table 1 . Detection of cytokine-producing antigen-specific T cells To investigate the ability of this assay to detect antigen-specific T-cell responses after stimulation with cognate antigen, we examined blood samples from HIV-infected subjects. PBMC were stimulated overnight with a HIV-Gag peptide pool, CMV lysate or Phorbol 12-myristate 13-acetate (PMA)/ionomycin, or left unstimulated. We then performed the flow-RNA assay to detect mRNA levels of IL-2 and IFNγ in the CD4 and CD8 T-cell subsets identified by the relevant surface markers. Results demonstrate that we can accurately identify cytokine mRNA-producing virus-specific CD4 T cells ( Fig. 3a–d ) and CD8 T cells ( Supplementary Fig. 3 ). In contrast to regular ICS where addition of Brefeldin and/or Monensin traps cytokines inside the cell for 6 to 12 h, leading to the accumulation of proteins produced over the duration of incubation; here, we detect an accurate ‘snapshot’ of mRNA expression at the specific time when the cells are fixed. Transcription and translation kinetics will also vary. Therefore, percentages of cytokine-producing cells after stimulation can differ between ICS and flow-mRNA assays. In spite of these differences, there was overall a good correlation between results when transcription (mRNA flow-FISH) and translation (ICS) of IFN-γ and IL-2 were examined in parallel ( Supplementary Fig. 4 ). The absence of cytokine secretion blockade in the flow-FISH approach is a significant advantage over standard ICS when cell–cell interactions are examined, as many cytokines work in autocrine and paracrine fashion to modulate activation signals. 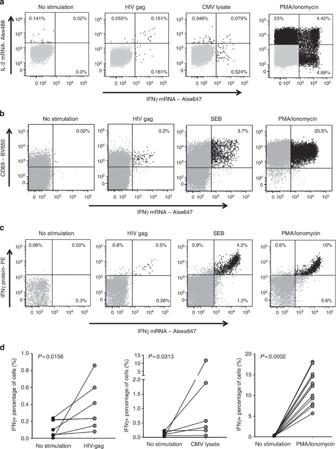Figure 3: IL-2 and IFNγ mRNA detection in antigen-specific CD4 T cells. (a) IL-2 and IFN-γ mRNA detection in CD4 T cells from PBMCs of an HIV-infected individual stimulated with a HIV-Gag peptide pool, CMV lysate or PMA/ionomycin for 12 h (one representative experiment out of five). (b) IFN-γ mRNA detection in combination with CD69 antibody staining from PBMCs of an HIV-infected subject left incubated with medium alone or stimulated with an HIV-Gag peptide pool, SEB or PMA/ionomycin for 12 h. (c) Combined detection of IFN-γ protein, using a 45 min capture assay, and IFN-γ mRNA in CD4 T cells from PBMCs of an HIV-infected person incubated with medium alone or stimulated with an HIV-Gag peptide pool, SEB or PMA/ionomycin for 12 h (one representative experiment out of five). (d) Collective data of IFN-γ mRNA detection after HIV-Gag peptide pool, CMV lysate or PMA/ionomycin stimulation. Statistical analysis was performed using a Wilcoxon matched-pairs test. Figure 3: IL-2 and IFNγ mRNA detection in antigen-specific CD4 T cells. ( a ) IL-2 and IFN-γ mRNA detection in CD4 T cells from PBMCs of an HIV-infected individual stimulated with a HIV-Gag peptide pool, CMV lysate or PMA/ionomycin for 12 h (one representative experiment out of five). ( b ) IFN-γ mRNA detection in combination with CD69 antibody staining from PBMCs of an HIV-infected subject left incubated with medium alone or stimulated with an HIV-Gag peptide pool, SEB or PMA/ionomycin for 12 h. ( c ) Combined detection of IFN-γ protein, using a 45 min capture assay, and IFN-γ mRNA in CD4 T cells from PBMCs of an HIV-infected person incubated with medium alone or stimulated with an HIV-Gag peptide pool, SEB or PMA/ionomycin for 12 h (one representative experiment out of five). ( d ) Collective data of IFN-γ mRNA detection after HIV-Gag peptide pool, CMV lysate or PMA/ionomycin stimulation. Statistical analysis was performed using a Wilcoxon matched-pairs test. Full size image To prove that the detection of mRNA is specific to activated cells, we utilized two different approaches. We first used an antibody against CD69, a surface molecule upregulated on most T cells on stimulation, in combination with mRNA detection. The large majority of IFN-γ mRNA+ cells were also CD69+, indicating specific detection of mRNA in the activated population ( Fig. 3b ). We next performed the flow-RNA assay in combination with a cytokine capture assay (Miltenyi Biotec, used per manufacturer’s instructions) that allows trapping of the molecule of interest by a primary antibody coated on the cell surface, followed by detection with a secondary fluorescent-labelled antibody. The IFN-γ capture phase lasts for 45 min and therefore stains cells that have secreted IFN-γ within this time frame. Figure 3c shows combined detection of IFN-γ protein by IFN-γ capture and mRNA production in HIV-specific T cells stimulated with HIV-Gag or T cells stimulated with Staphylococcal enterotoxin B (SEB) or PMA. These data show overall very good consistency; however, after SEB and PMA/ionomycin stimulation we observed a small percentage of cells harbouring IFNγ mRNA but on which no IFN-γ protein was detected by the capture assay: about 20% of the CD4 T cells expressing IFNγ mRNA on SEB stimulation and 35% of the CD4 T cells expressing IFNγ mRNA on PMA stimulation were negative by IFNγ capture. This difference may be due to both a difference in sensitivity as well as different in kinetics with a delay between transcription and translation. These data show that the flow-RNA assay is sensitive enough to detect antigen-specific T cells and can be used to detect cytokine transcription and translation in the same cells, which can be very useful for studies of functional regulation of immune cells. Sensitive detection of molecules with poor antibody staining One of the major limitations of antibody-based flow cytometry is that although thousands of suitable antibodies are commercially available, these still do not cover the full panel of molecules of interest present within a cell. Moreover, antibodies have variable sensitivities and often do not perform well at detecting weakly expressed antigens. Flow-RNA offers the potential to stain for a much more diverse selection of molecules. To test this, we first decided to stain for the cytokine IL-21, as the low sensitivity of its detection by ICS has been a hurdle for many investigators. IL-21 is a cytokine critical for CD4 T cell help to B cells and CD8 T cells, but is also implicated in several autoimmune diseases [19] , including idiopathic thrombocytopenic purpura (ITP). ITP is characterized by abnormal production of antibodies that attack platelets. These autoantibodies have been linked to abnormal T follicular helper cells that produce increased amounts of IL-21 (ref. 20 ). We thus decided to test the ability of the mRNA-FISH assay to detect IL-21 compared with ICS in spleen mononuclear cell samples from two subjects that had undergone splenectomy for ITP refractory to medical treatment and from one individual who had surgery for traumatic splenic rupture. Despite maximal stimulation with PMA/ionomycin, ICS assays on splenocytes detected only small levels of IL-21 protein in all three subjects investigated ( Fig. 4 ), whereas robust production of IL-2 was identified. In contrast to ICS, the mRNA flow-FISH assay was able to detect a much greater percentage of IL-21-secreting cells after PMA/ionomycin stimulation, whereas the fraction of IL-2-secreting CD4 T cells was overall similar with the two techniques. Interestingly, this massive production of IL-21 was present in the two ITP subjects ( Fig. 4a,b ) but very low in the control sample ( Fig. 4c ). Extension of these experiments to five additional subjects who underwent splenectomy for indications unrelated to hematologic or autoimmune disorders confirmed low IL-21 mRNA expression compared to individuals with ITP ( Fig. 4d ). Detection of IL-21 mRNA was restricted to CD4 T cells and not CD8 T cells ( Supplementary Fig. 5 ), consistent with the known role of CD4 T cells as the main producers of IL-21. We were able to simultaneously use three different probes to detect mRNA levels of IL-2 (Alexa 488), IL-21 (Alexa 647) and IFN-γ (Alexa 750) in CD4 T cells from these patients ( Supplementary Fig. 6 ), allowing for detailed investigation of co-expression patterns at the single-cell level. 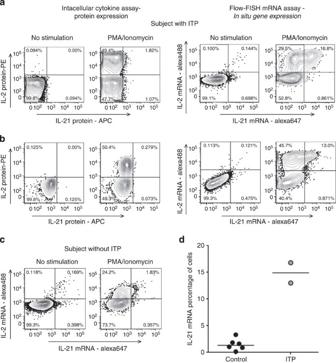Figure 4: Detection of IL-21 mRNA in CD4 T cells. Lymphocytes isolated from a spleen sample of two subjects suffering from ITP (a,b) and one subject who underwent surgery for traumatic splenic rupture (c). Cells were incubated with culture medium alone or stimulated overnight with PMA/ionomycin, with addition of brefeldin and monensin only for the ICS assay. Following incubation, cells were stained either following a standard ICS protocol or with the new flow-RNA-FISH protocol for dead cell dye, surface lineage markers and either cytokine-specific antibodies or cytokine-specific probe sets. (d) Collective data on IL-21 mRNA expression after PMA/ionomycin stimulation in CD4 T cells from six negative control and two ITP subjects. Figure 4: Detection of IL-21 mRNA in CD4 T cells. Lymphocytes isolated from a spleen sample of two subjects suffering from ITP ( a , b ) and one subject who underwent surgery for traumatic splenic rupture ( c ). Cells were incubated with culture medium alone or stimulated overnight with PMA/ionomycin, with addition of brefeldin and monensin only for the ICS assay. Following incubation, cells were stained either following a standard ICS protocol or with the new flow-RNA-FISH protocol for dead cell dye, surface lineage markers and either cytokine-specific antibodies or cytokine-specific probe sets. ( d ) Collective data on IL-21 mRNA expression after PMA/ionomycin stimulation in CD4 T cells from six negative control and two ITP subjects. Full size image We next decided to investigate expression of an enzyme for which there was no commercially available antibody for flow cytometry at the time that this experiment was performed, IDO. An antibody detecting intracellular IDO became recently available (eBioscience). IDO is critical for metabolism of tryptophan, an essential amino acid. Catabolism of tryptophan by IDO results in an immunosuppressive environment that has been implicated in the pathogenesis of cancer, autoimmunity and chronic infections [21] , [22] . Stimulation of PBMCs with the TLR7/8 agonist ligand R848 or with combination of IFN-γ and lipopolysaccharide (LPS) for 8 h led to robust upregulation of IDO mRNA in monocytes ( Fig. 5a,b ). We also found a strong correlation between IDO mRNA expression in CD14+ cells by flow-FISH and the relative mRNA levels as measured by quantitative reverse transcription–PCR (qRT–PCR; Fig. 5c ), These data show the unique capacity of the flow-FISH assay to detect mRNA expression of molecules that cannot be detected with antibody-based flow cytometry. 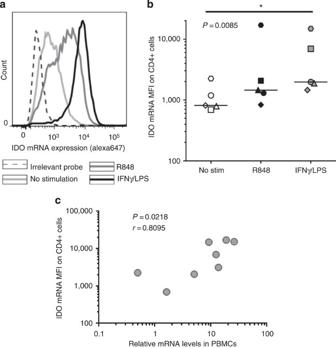Figure 5: Detection of IDO in monocytes. PBMCs from an HIV-negative subject were stimulated for 8 h with either R848 or IFNγ+LPS. IDO mRNA detection in monocytes was achieved after gating on the CD14 positive cell subset within the monocyte gate. (a) Representative example and (b) collective data on five different subjects. Statistical analysis used Friedman test with a Dunn’s post-test comparison. (c) Correlation between IDO mRNA mean fluorescent intensity (MFI) in CD14+ cells and IDO relative mRNA expression as measured by qPCR in PBMCs from the same experiment. Statistical analysis used the Spearman rank sum test. Figure 5: Detection of IDO in monocytes. PBMCs from an HIV-negative subject were stimulated for 8 h with either R848 or IFNγ+LPS. IDO mRNA detection in monocytes was achieved after gating on the CD14 positive cell subset within the monocyte gate. ( a ) Representative example and ( b ) collective data on five different subjects. Statistical analysis used Friedman test with a Dunn’s post-test comparison. ( c ) Correlation between IDO mRNA mean fluorescent intensity (MFI) in CD14+ cells and IDO relative mRNA expression as measured by qPCR in PBMCs from the same experiment. Statistical analysis used the Spearman rank sum test. Full size image miRNA detection in primary T cells by flow cytometry We next utilized this technique to detect miRNA expression in primary T cells after PMA/ionomycin stimulation. miRNAs are small non-coding RNAs that control gene expression at the post-transcriptional level and play a critical role in regulating cell functions. Here we used flow-FISH to detect two miRNA targets, miR-21 and miR-155 that have been shown to control immune responses [23] , [24] . Stimulation of CD4 and CD8 T cells for 12 h did not significantly enhance miR-21 expression but led to increased expression of miR-155 ( Fig. 6 ). This is consistent with the literature that showed miR-155 to be one of the few miRNA upregulated in T cells after stimulation, whereas miR-21 is not significantly enhanced [25] . miRNA expression was measured in activated CD69+ CD4 ( Fig. 6d ) and CD8 T cells ( Fig. 6c ) proving the ability of flow-RNA to provide insight into single-cell co-expression of miRNAs in combination with mRNAs molecules and proteins of interest. These data show the unprecedented capabilities of this novel method to also quantify small non-coding miRNA molecules that act as critical regulators of mRNA translation. 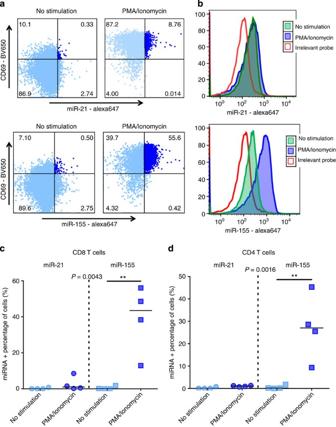Figure 6: miRNA detection in CD4 and CD8 T cells with flow cytometry. PBMCs from HIV-negative subjects were left unstimulated or were stimulated overnight with PMA/ionomycin. (a,b) Representative example of miR-21 and miR-155 expression in CD8 T cells. (c,d) Collective data on four subjects for the detection of miR-21 and miR-155 in CD69+activated CD8 and CD4 T cells. Statistical analysis used Friedman test with a Dunn’s post-test comparison. Figure 6: miRNA detection in CD4 and CD8 T cells with flow cytometry. PBMCs from HIV-negative subjects were left unstimulated or were stimulated overnight with PMA/ionomycin. ( a , b ) Representative example of miR-21 and miR-155 expression in CD8 T cells. ( c , d ) Collective data on four subjects for the detection of miR-21 and miR-155 in CD69+activated CD8 and CD4 T cells. Statistical analysis used Friedman test with a Dunn’s post-test comparison. Full size image Combined mRNA and protein visualization using ImageStream One of the disadvantages of any traditional flow cytometry technique compared with microscopy is that one cannot visualize subcellular localization of molecules. The newly developed ImageStream technology (Amnis) combines the advantages of high-throughput flow stream analyses with microscopy capabilities. Although not reaching the spatial definition of standard fluorescent microscopy, this platform allows much easier acquisition of statistically significant cell numbers in heterogeneous populations. Developing combined detection of multiple mRNAs and proteins with this technology thus has the potential of considerably expanding the versatility of its applications. To assess the applicability of the flow-RNA protocol to the ImageStream platform, we again used a cytokine protein capture assay combined with cytokine mRNA quantitation. We were able to simultaneously detect IFN-γ protein and IFN-γ mRNA in blood CD4 T cells from a healthy subject ( Fig. 7 ). These data show the potential application of flow-RNA to perform ImageStream experiments for high-throughput co-vizualization of mRNA, miRNA and protein at the single-cell level and briefly demonstrate the potential for flow-FISH in co-localization studies. This approach may be applied to investigations of cellular localization in protein–mRNA or miRNA–target mRNA interaction studies. 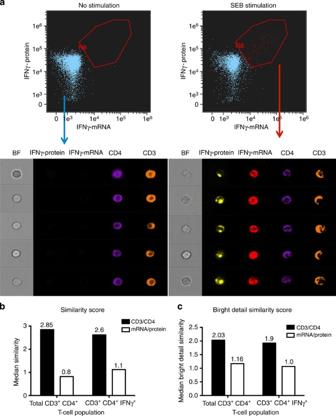Figure 7: Combined detection of IFNγ protein and mRNA with ImageStream. (a) PBMCs from an HIV-negative subject were left unstimulated or stimulated with SEB for 12 h. At the end of this incubation time, a 45-min capture assay was performed for detection of IFNγ-protein, followed by IFN-γ mRNA staining with the flow-FISH assay. CD4 T cells were then acquired on an ImageStream instrument. Images illustrate expression of IFN-γ protein, IFN-γ mRNA, CD4 and CD3 in the lymphocyte gate in unstimulated cells (left panels) and in stimulated cells (right panels). (b,c) Co-localization analysis for CD3/CD4 in black and IFNg protein/mRNA in white using two different analytical tools (b) Similarity score (the log-transformed Pearson’s correlation coefficient, measuring the spatial linear correlation between two total stains within a cell mask) and (c) Bright detail similarity score (the log-transformed Pearson’s correlation coefficient, measuring the spatial linear correlation between the only the bright regions of two stains within a cell mask). We found a low correlation between secreted IFNg protein and internal mRNA using both measures (median score ~1). In comparison, surface stained CD3 and CD4 were well correlated (median score ~2). Figure 7: Combined detection of IFNγ protein and mRNA with ImageStream. ( a ) PBMCs from an HIV-negative subject were left unstimulated or stimulated with SEB for 12 h. At the end of this incubation time, a 45-min capture assay was performed for detection of IFNγ-protein, followed by IFN-γ mRNA staining with the flow-FISH assay. CD4 T cells were then acquired on an ImageStream instrument. Images illustrate expression of IFN-γ protein, IFN-γ mRNA, CD4 and CD3 in the lymphocyte gate in unstimulated cells (left panels) and in stimulated cells (right panels). ( b , c ) Co-localization analysis for CD3/CD4 in black and IFNg protein/mRNA in white using two different analytical tools ( b ) Similarity score (the log-transformed Pearson’s correlation coefficient, measuring the spatial linear correlation between two total stains within a cell mask) and ( c ) Bright detail similarity score (the log-transformed Pearson’s correlation coefficient, measuring the spatial linear correlation between the only the bright regions of two stains within a cell mask). We found a low correlation between secreted IFNg protein and internal mRNA using both measures (median score ~1). In comparison, surface stained CD3 and CD4 were well correlated (median score ~2). Full size image Fluorescent in situ hybridization (FISH) enables the detection of nucleic acid sequences at the single-cell level. Until now, this powerful technology has been largely limited to fluorescent microscopy imaging, thus limiting its use for analysis of heterogeneous cell populations, which require acquisition of large numbers of events. Even though a number of attempts have been made to adapt this method to flow cytometry, they overall showed reduced sensitivity, often relatively poor specificity, time-consuming experimental design and lack of versatility with different nucleic acid targets requiring individualized protocols. Critically, they did not allow simultaneous detection of multiple targets in the same sample, and were hampered by the lack of compatibility between RNA-FISH and antibody staining for cell surface markers. Here we show the application of a novel, powerful RNA-FISH technology in various optimized flow cytometry protocols that overcome several significant hurdles toward the study of cell function, gene expression and transcriptional regulation in heterogeneous cell samples. The approach presented here is derived from reagents initially developed for fluorescent microscopy (QuantiGene ViewRNA) that have been successfully used to detect DNA, mRNA and miRNAs sequences [17] . Direct application of the QuantiGene ViewRNA protocol to PBMC samples was accompanied by severe cell loss. Furthermore, addition of protease, which enhances accessibility of probes to their target, resulted in poor antibody staining for cell surface markers, probably because of alteration in antigen conformation. We therefore made use of a new protocol using a methanol-based permeabilization step. We show here that this procedure is compatible with dead cell dyes and, critically, antibody staining for a variety of cell surface proteins. The depth of data provided is thus similar to standard polychromatic flow cytometry. Reagents currently available allow multiplexing for three different sets of probes for the fluorochromes Alexa 488, 647 and 750. The method is compatible with a wide array of small-molecule dyes such as Brilliant Violet, Alexa dyes and eFluors, but not with protein-based fluorescent dyes, such as PE, PerCP and APC, and their tandem dye conjugates. Methanol is also known to denature some epitopes, such that some monoclonal antibodies are necessarily incompatible with this method. After having optimized hybridization times and combination of mRNA probes, surface antibody staining and dead cell dye, we applied the protocol to PMBCs isolated from HIV-infected individuals. We were able to accurately identify CD4 and CD8 T cells and to detect mRNA expression for the cytokines IFN-γ and IL-2 by HIV- and CMV-specific T cells after cognate antigen stimulation, with sensitivity comparable to standard ICS for the corresponding cytokine proteins. This mRNA upregulation was exclusively observed within CD69+ cells, confirming that it occurred on activation. To compare transcription and translation levels of the same cytokine, we were next able to combine an IFN-γ capture assay that traps secreted proteins on the cell surface with mRNA detection. Besides further confirming the validity of the assay, we believe that this combined assay opens up interesting possibilities to study regulation of cytokine or chemokine production in mixed populations of immune cells. Depending on the question to be addressed, combination with the capture assay can also overcome one current limitation of the mRNA-FISH assay, which is its incompatibility with intracellular staining for proteins. Technically, this limitation can probably be overcome by modification of the fixation and permeabilization procedures, but this will require further investigation. A major strength of this assay is the potential to detect many mRNAs of interest without being limited by antibody availability. This has great applicability for studies on animal species for which antibody availability for flow cytometry is limited. All FISH probes are derived by an algorithm that enables them to have similar hybridization temperatures and therefore allows combination of different probes and reproducibility between different assays. We were able to detect a combination of three different probes for the cytokines IL-2, IL-21 and IFN-γ in the same sample, highlighting the unique multiplexing ability of this method. Besides the large panel of ready-made probes available, custom-designed probes can also be ordered for the gene of interest. We also assessed the ability of the flow-RNA assay to detect expression of mRNAs for which detection with antibody is either poor or not available. Detection of IL-21 mRNA was clearly superior to identification of IL-21 protein by standard ICS assay. The potential significance of this finding is illustrated by our results on spleen samples from two subjects with ITP, an autoimmune disease in which IL-21 is known to play a role. Whereas ICS revealed little, we found a marked upregulation of IL-21 transcription in CD4+ splenocytes on stimulation in these patients, contrasting with low induction in six subjects with no underlying autoimmune disorder. This technique can thus be used to define altered gene expression patterns in primary cells in the context of human diseases. We could also clearly detect the upregulation of transcription of the immunomodulating enzyme IDO in monocytes after stimulation with TLR agonists, whereas no antibody was commercially available to detect IDO by flow cytometry at the time of these experiments. Recently, it has become increasingly clear that non-coding RNAs, including miRNAs and long non-coding RNAs, play broad and critical regulatory roles in cell regulation, including immune responses. We thus also investigated the ability of mRNA flow-FISH to detect such nucleic acids sequences for which there is no protein translation. miRNAs control gene expression at the post-transcriptional level by translational repression or enhanced target degradation. In spite of the short sequence of miRNAs (around 22 nucleotides), we successfully detected miR-155 modulation in CD4 and CD8 T cells after stimulation. The implication of miRNAs in many diseases makes them attractive targets for immunotherapeutic interventions and biomarker development for cancer and autoimmune diseases [26] , [27] . Our proof-of-principle experiments indicate the unprecedented capabilities of this assay to simultaneously detect expression of miRNA, mRNA and protein at the single-cell level, providing a tool for in-depth analysis of miRNA function in combination with their translational and expressional effects in both normal and pathologic conditions. As flow cytometry does not show localization of protein expression within cells, we finally explored the potential of the flow-RNA assay to be used with ImageStream technology. We successfully detected IFN-γ mRNA and protein levels on CD4 T cells after SEB stimulation, with excellent signal/noise ratios for the different parameters measured. Thus, this assay can be used with this novel instrument combining some of the advantages of both polychromatic flow cytometry and fluorescent microscopy, including compartmentalization studies. In conclusion, this novel mRNA/miRNA flow-FISH assay presents major advantages over previous technologies including: an algorithm-based controlled design of probes that allows reproducibility and combination of various probes with similar hybridization conditions; the straightforward combination with fluorescent antibody staining that allows simultaneous phenotyping of heterogeneous cell populations; the design of probes for molecules for which no antibody is available; the user-friendly protocol that has many similarities with standard antibody staining procedures for regular flow cytometry; and the processing and data acquisition with standard laboratory equipment and cytometers. Our data illustrate the versatility of this technique and its broad applicability for analysis of normal cell functions and disease states. Human subjects Peripheral blood was obtained from HIV-infected and uninfected individuals at the Massachusetts General Hospital (MGH), Boston. The study was approved by the MGH Institutional Review Board and written informed consent was obtained from all study participants before enrolment in the study. PBMCs were isolated by Ficoll density centrifugation. Frozen PBMCs were thawed and were cultured in RPMI 1640 medium (Invitrogen) supplemented with HEPES, penicillin, streptomycin and 10% human AB serum (Gemini Bioproducts) (R10 medium). Non-identifiable excess spleen tissue was obtained at Massachusetts General Hospital under approval by the Partners Human Resource Committee. These surgeries were performed for medical or surgical indications not related to hematologic or autoimmune diseases, with the exception of two patients who underwent splenectomy for refractory ITP, which is currently an uncommon indication for such an intervention. Spleens were dissected into small fragments and subsequently mechanically disrupted to single-cell suspension using a 70-μm cell strainer and a syringe plunger. Following washing in R10 medium containing 2 mM EDTA, cells were strained once more and erythrocytes were lysed using RBC lysis buffer (Qiagen). Cells were immediately cryopreserved for subsequent use. Cell stimulation Cells were resuspended in 500 ul R10 medium before being stimulated with an HIV-Gag peptide pool (2 μg ml −1 per peptide), CMV lysate (1 μg ml −1 ), SEB (1 μg ml −1 ), PMA/ionomycin (1 × , Cell Stimulation Cocktail, eBioscience), TLR7/8 agonist R848 (10 ng ml −1 ) or recombinant IFNγ (100 ng ml −1 )+LPS (10 ng ml −1 ). Flow-FISH method PBMCs were stained with viability dye (Invitrogen LIVE/DEAD) for 30 min at room temperature. Surface antibodies were then added to stain for cell populations of interest (BV711 CD3 (5 μl per 100 μl of sample, clone: OKT3), BV421 CD4(5 μl per 100 μl of sample, clone: OKT4), V500 CD8 (5 ul per 100 μl of sample, clone: SK1) and BV605 CD14 (5 μl per 100 μl of sample, clone: M5E2)). Assay was performed as per manufacturer’s instructions (Affymetrix, Inc., http://media.ebioscience.com/data/pdf/literature/quantigene-flowrna-user-manual.pdf ). In brief, PBMCs were fixed with a 4% paraformaldehyde solution for 1 h at room temperature. Cells were then permeabilized with ice-cold methanol, followed by further fixation with a 4% paraformaldehyde solution for 30 min at room temperature. All buffers used in the following steps were included in the manufacturer’s kit. To detect mRNA, probes comprised of ~20 oligonucleotide base pairs against the mRNA of interest were used. Currently, there are three different types of probes with unique tag sequences, named type 1, type 4 and type 6, respectively. Each tag sequence allows the hybridization of specific complementary branched DNA nanostructure with different excitation/emission spectra: type 1–650/668, type 4–495/519 and type 6–749/775. Probes were diluted 1:20 in target probe diluent, added to the cell suspension and allowed to hybridize to the target RNA for 2 h at 40 °C. Excess probe was removed by adding wash buffer followed by centrifugation at 800 g for 5 min. Signal amplification was achieved by performing sequential hybridization with DNA branches (that is, Pre-Amplifier and Amplifier). The first DNA branch in the PreAmp Mix was added at a 1:1 ratio and was allowed to hybridize for 1.5 h at 40 °C. Samples were washed with wash buffer, and then the second DNA branch in the Amp Mix was added at a 1:1 ratio and hybridized for 1.5 h at 40 °C. Samples were washed with wash buffer before addition of the label probes. For signal detection, fluorochrome-conjugated label probes were diluted 1:100 in label probe diluent, added to the samples and allowed to hybridize for 1 h at 40 °C. Finally, PMBCs were washed with wash buffer, transferred to the storage buffer and subsequently analysed on a LSR Fortessa, using FACS DIVA software version 7 (BD Biosciences, San Jose CA). Flow cytometric data were analysed with FlowJo Version 7.5.5 (TreeStar). As negative controls, we used probes that target irrelevant sequences for dihydrodipicolinate reductase/dapB gene of the bacterium Bacillus subtilis that should not be encountered in human samples. For the experiments where alterations of mRNA levels were investigated after stimulation, the gates were set according to the unstimulated control. Optimization of target probe hybridization time To determine the optimal hybridization time in terms of the signal-to-noise ratio, we varied the target probe hybridization times from 1 to 4 h. Both a negative control probe, dapB ( Bacillus subtilis ), and a probe for housekeeping gene β2-microglobulin (type 1 probe) were used. mRNA detection in activated CD4 T cells PBMCs were either left unstimulated or were stimulated with HIV-Gag, SEB or PMA/ionomycin overnight (16 h). The next day, cells were stained with viability dye and a panel of surface antibodies ((CD3-BV711 (5 μl per 100 μl of sample, clone: OKT3), CD4-BV421(5 μl per 100 μl of sample, clone: OKT4), CD8-BV605 (5 μl per 100 μl of sample, clone: RPA-T8), CD14-V500 (5 μl per 100 μl of sample, clone: M5E2 and CD69-BV650(5 μl per 100 μl of sample, clone: FN50)). The flow-FISH protocol was followed as outlined above, and IFNγ mRNA type 4 probes were detected in activated CD4 T cells (CD4+/CD69+) on the LSR Fortessa ( Fig. 2b ). For detection of IL-21 CD4 T cells from spleen samples of subjects with ITP, we stimulated cells for 12 h with PMA/ionomycin. The flow-FISH protocol was followed as outlined above, and IL-2 (type 4 probes), IL-21 (type 1 probes) and IFNγ (type 6 probes) mRNA on CD4 and CD8 T cells were measured on a BD Fortessa ( Fig. 3 ). We also performed ICS from the same samples to compare IL-21 detection between ICS and the new flow-FISH protocol. In brief, cells were stimulated with PMA/ionomycin for 12 h in the presence of Monensin and Brefeldin A (5 μg ml −1 ). Subsequently, cells were stained with blue viability dye (Invitrogen Life Technologies) and fluorescent antibodies against CD3 (5 μl per 100 μl of sample, clone: OKT3), CD4(5 μl per 100 μl of sample, clone: OKT4), CD8 (5 ul per 100 μl of sample, clone: SK1), CD14 (5 μl per 100 μl of sample, clone: M5E2) and CD19 (5 μl per 100 μl of sample, clone: HIB19). Intracellular staining for IFNγ, IL-2 and IL-21 was performed using BD Cytofix/Cytoperm Fixation/Permeabilization Solution according to the manufacturer’s instructions. Cells were then analysed on the LSR Fortessa. Simultaneous detection of cytokine mRNA and protein To determine whether the mRNA we were detecting correlated with the cells producing the protein, PBMCs were stimulated overnight with either HIV-Gag peptide pools, SEB or PMA/ionomycin. Cells were then labelled with IFNγ catch reagent using the Miltenyi IFN γ capture assay kit and protocol. Cells were allowed to secrete cytokines for 45 min before commencing staining. Cells were stained with viability dye and surface antibodies (CD3-BV711 (5 μl per 100 μl of sample, clone: OKT3), CD4-BV421 (5 μl per 100 μl of sample, clone: OKT4), CD8-V500 (5 ul per 100 μl of sample, clone: SK1) and CD69-BV650 (5 μl per 100 μl of sample, clone: FN50)), and the flow-FISH was followed. After completing washes outlined at the end of the protocol, cells were labelled with anti-IFN γ PE detection reagent following the Miltenyi protocol. The PE detection reagent was added after the flow-FISH protocol was completed because, if added before the fixation and permeabilization steps, the methanol would have degraded the protein dye and no IFN γ protein signal would have been observed. Cells were then analysed on the LSR Fortessa. IDO mRNA detection with Flow-FISH and qRT–PCR PBMCs from HIV-negative subjects were stimulated with R848 or IFNγ+LPS for 8 h. After 8 h, the cells were split into two, and half of them were processed with the flow-FISH assay for detection of IDO mRNA (type 4 probe) on CD14 cells (CD3-BV711 (5 μl per 100 μl of sample, clone: OKT3), CD19-V500 (5 μl per 100 μl of sample, clone: HIB19) and CD14-BV605 (5 μl per 100 μl of sample, clone: M5E2)) and the other half was lysed in RLT buffer containing 1% beta-mercaptoethanol followed by mRNA extraction with the Qiagen mRNA isolation kit. qRT–PCR for IDO and GAPDH housekeeping gene was performed using Taqman probes from ABI according to the manufacturer’s instructions. Detection of miRNA with flow-FISH PBMCs from HIV-negative subjects were either left unstimulated or were stimulated for 12 h with PMA/ionomycin. Flow-FISH protocol was followed as described above. Probes specific for miR-21 and miR-155 (type 1) were used. Cells were stained with surface antibodies (CD3-BV711 (5 μl per 100 μl of sample, clone: OKT3), CD4-BV421 (5 μl per 100 μl of sample, clone: OKT4), CD8-V500 (5 ul per 100 μl of sample, clone: SK1) and CD69-BV650 (5 μl per 100 μl of sample, clone: FN50)) and miRNA probes were detected in activated CD4 T cells (CD4+/CD69+) on a LSR Fortessa. Imaging flow cytometry to visualize mRNA and protein To visualize simultaneous detection of IFN γ mRNA and protein PBMCs were left unstimulated or were stimulated with SEB for 12 h. Flow-FISH in combination with the IFNγ capture assay were performed as described above. For each sample, 30,000 cells were collected on a five-laser two-camera ImageStream Mark II imaging flow cytometer (Amnis, Seattle, WA). This instrument combines the immunofluorescent sensitivity and capacity of a traditional flow cytometer with bright-field high-resolution microscopy and image analysis. Since the ImageStream has an alternate excitation capacity than the LSR Fortessa, alternate antibody fluorochrome conjugates were necessary to achieve optimal detection. For this reason, we used CD8-BV785 (5 μl per 100 μl of sample, clone: RPA-T8), CD3-BV605 (5 μl per 100 μl of sample, clone: OKT3) and CD4-BV421 (5 μl per 100 μl of sample, clone: OKT4). Images were captured with INSPIRE acquisition software (Amnis v.6.0.154.0) utilizing × 40 magnification. Post-acquisition data analysis was performed using IDEAS software (Amnis v.6.0.333.0). Single, focused cells were gated using Gradient RMS (focus), then Area versus Aspect Ratio in the Bright-field (BF) channel. Next, CD3+ events were gated based on Intensity (versus BF area). From the CD3+ population, a bivariate intensity plot of CD4 versus CD8 was generated to gate the CD8+ population. How to cite this article: Porichis, F. et al. High-throughput detection of miRNAs and gene-specific mRNA at the single-cell level by flow cytometry. Nat. Commun. 5:5641 doi: 10.1038/ncomms6641 (2014).